A CO2electrolyzer tandem cell system for CO2-CO co-feed valorization in a Ni-N-C/Cu-catalyzed reaction cascade Coupled tandem electrolyzer concepts have been predicted to offer kinetic benefits to sluggish catalytic reactions thanks to their flexibility of reaction environments in each cell. Here we design, assemble, test, and analyze the first complete low-temperature, neutral-pH, cathode precious metal-free tandem CO 2 electrolyzer cell chain. The tandem system couples an Ag-free CO 2 -to-CO 2 /CO electrolyzer (cell-1) to a CO 2 /CO-to-C 2+ product electrolyzer (cell-2). Cell-1 and cell-2 incorporate selective Ni-N-C-based and Cu-based Gas Diffusion Cathodes, respectively, and operate at sustainable neutral pH conditions. Using our tandem cell system, we report strongly enhanced rates for the production of ethylene (by 50%) and alcohols (by 100%) and a sharply increased C 2+ energy efficiency (by 100%) at current densities of up to 700 mA cm −2 compared to the single CO 2 -to-C 2+ electrolyzer cell system approach. This study demonstrates that coupled tandem electrolyzer cell systems can offer kinetic and practical energetic benefits over single-cell designs for the production of value-added C 2+ chemicals and fuels directly from CO 2 feeds without intermediate separation or purification. In the light of intensified efforts to mitigate power and chemicals production from fossil sources and their substitution by renewable ones, electrocatalytic power-to-chemicals and power-to-fuels technologies are emerging as one of the future pillars of sustainable chemicals industry [1] . Recent years have seen a drastic increase in attention for the electrocatalytic CO 2 reduction reaction (CO 2 RR), advancing the production of 2e − reduction products, such as CO and formic acid , towards commercialization [2] , [3] , [4] . In contrast, the electrocatalytic reaction process pathway towards C 2+ hydrocarbons and oxygenates, in particular C 2 H 4 , Ethanol, Propanol, lacks similar technological advances [5] , [6] , [7] , [8] , [9] , [10] . Following Hori’s pivotal work on CO 2 RR, establishing CO as key intermediate in hydrocarbons and oxygenates production, studies investigated CO as feedstock in what is referred to as the CO reduction reaction (CORR). CORR achieves a higher faradaic efficiency (FE) for the production of C 2+ compounds, in part because some common C 1 side-products of the CO 2 RR, such as CO or HCOO - , cannot be formed, but also due to more favorable kinetics and surface coverages of H * and CO * . Specifically, the production of oxygenates has been shown to be favored by CORR compared to CO 2 RR, especially under alkaline conditions that are only sustainable for CORR due to the invariable formation of (bi)carbonate from CO 2 [11] , [12] , [13] , [14] , [15] , [16] , [17] , [18] , [19] . The favorable kinetics of alkaline CORR compared to CO 2 RR for production of C 2+ species has motivated researchers to try to find ways to separate off the CORR in a CO 2 RR electrolyzer. Tandem Cathode Concepts follow the idea to spatially decouple the initial 2e - reduction of CO 2 to CO and the subsequent reduction steps of CO towards C 2+ products. The tandem split can be realized at vastly different length scales and distinct configurations: (i) at the atomic scale by two neighboring active sites coupled by CO spillover, (ii) at the macroscopic electrode scale with macroscopically separated regions of distinct catalysts inside the same electrolyzer cell, and (iii) at the macroscopic electrolyzer cell scale forming a coupled process cascade [20] , [21] , [22] , [23] , [24] , [25] , [26] , [27] , [28] , [29] , [30] , [31] , [32] , [33] , [34] , [35] . While the idea of placing the active sites of CO source and sink inside the same electrode is an intriguing one, it has been shown to be inherently sensitive to the relative spatial catalyst distribution that is challenging to maintain over longer operation times considering the reported mobility of Cu catalysts under CO 2 RR [36] , [37] , [38] , [39] , [40] , [41] . The present work sets out to explore the coupled tandem electrolyzer cell approach, i.e., two individual electrolyzers in series, for a significantly enhanced production of C 2+ compounds from CO 2 in a catalytic reaction cascade. We deliberately avoid the use of high-temperature technologies, harsh reaction conditions, and demonstrate the advantages by avoiding CO 2 scrubbing steps to increase the practicality of the overall process, and make use of kinetic benefits for CO 2 /CO co-feeds agreeing with the presence of reactant- and product-specific reaction sites on Cu catalysts [20] , [42] . Accordingly, we deploy a noble metal-free single Ni atom site electrocatalyst (Ni-N-C) in a neutral-pH, near-ambient temperature, zero-gap setup for selective conversion of CO 2 to CO-rich CO 2 /CO mixed streams. The CO 2 /CO mixed feed was then directly introduced to a second flow electrolyzer cell equipped with a Cu-catalyst for conversion of CO 2 /CO mixed feeds into C 2+ products. We report strongly enhanced rates for the production of ethylene (~50%) and of alcohols (>= 100%) and a sharply increased C 2+ energy efficiency (>=100%) in the tandem systems compared to the conventional single CO 2 electrolyzer cell approach. To validate our conclusions and provide kinetic insight, we also conducted single-cell control experiments with controlled mixed CO 2 /CO co-feeds to explore the origin of the observed tandem effect. These experiments suggest that CO 2 is being selectively scrubbed from the gas mixture by cathodically generated OH - in vicinity of the cathode thus locally increasing the effective CO concentration and CO surface coverage, mimicking the performance of CO-rich gas feeds. 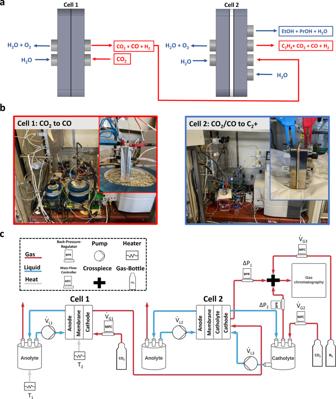Fig. 1: Illustration of the tandem electrolyzer cell system used for efficient CO2valorization. aConcept of coupled Tandem CO2Electrolyzer Cells highlighting the flows of gas (red) and liquid (blue) reactants and products. Additional information on the detailed reaction conditions can be found in Supplementary Fig.2.bPhotographs of the two electrolysis reactors used for coupled CO2-to-CO electrolysis and CO2/CO-to-C2+electrolysis, with inserts showing an enlargement of the cells used in each case.cDetailed Process scheme of tandem cell set up with information on gas (red) and liquid (blue) flow directions and the most important components of the investigated tandem system. Design of a low-temperature tandem electrolyzer cascade for the production of C 2+ compounds Figure 1a introduces the concept and the process design of the first low-temperature coupled tandem CO 2 electrolyzer cell system developed and studied in this contribution. Fig. 1: Illustration of the tandem electrolyzer cell system used for efficient CO 2 valorization. a Concept of coupled Tandem CO 2 Electrolyzer Cells highlighting the flows of gas (red) and liquid (blue) reactants and products. Additional information on the detailed reaction conditions can be found in Supplementary Fig. 2 . b Photographs of the two electrolysis reactors used for coupled CO 2 -to-CO electrolysis and CO 2 /CO-to-C 2+ electrolysis, with inserts showing an enlargement of the cells used in each case. c Detailed Process scheme of tandem cell set up with information on gas (red) and liquid (blue) flow directions and the most important components of the investigated tandem system. Full size image The numbering of the cells refers to the order in which they were deployed in the tandem system electrolyzer cascade and is used as a denomination throughout this work. Cell-1, the first electrolyzer in the reaction cascade, converts CO 2 to CO and is the point of entry for the CO 2 feed. At the cathode Gas Diffusion Electrode (GDE) of cell-1, we use a previously developed noble metal-free single Ni atom site electrocatalyst (NiNC) deployed into a neutral anode-pH, zero-cathode-gap electrode design [43] . Since the stoichiometric CO 2 ratio, λ stoich , remains above one, the cathodic CO 2 to CO conversion in cell-1 invariably results in mixed CO 2 /CO exit feeds, even if the cathode is operated at 100% faradaic CO efficiency. This mixed CO 2 /CO gas feed is directly used as input feed for a Cu-based electrolyzer “cell-2” to efficiently produce C 2+ products, as schematically depicted in Fig. 1a . Note, that while within this work we refer to the commercial Cu catalysts as “Cu” for simplicity, XRD analysis showed that the material is partially oxidized and shows a presence of a Cu 2 O phase, see Supplementary Fig. 1 . Figure 1b shows photographs of our experimental setup with inserts of the individual electrolysis cells used during electrochemical characterization. The detailed tandem cell process scheme is given in Fig. 1c . Note how cell-1 and cell-2 were connected in series by the CO 2 gas flow to enable an enrichment with CO in the gas stream before entering cell-2. A more detailed discussion on the geometry of the individual cells and testing setup including operational parameters can be found in Supplementary Fig. 2 . Electrochemical CO 2 /CO mixed gas feed reduction Prior to coupled tandem electrolyzer cell experiments, we studied how the presence of CO in the CO 2 reactant gas feed affects the product production rates of a single Cu cathode-based CO 2 electrolyzer. 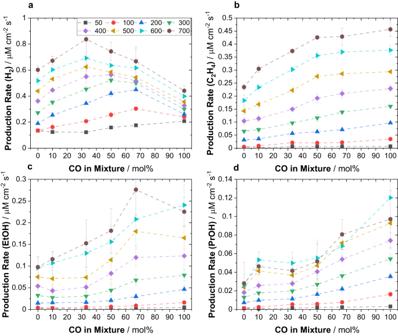Fig. 2: Influence of CO2/CO co-feed composition on production rates observed for electrolysis in single-cell experiments of cell-2. Production rates of key products using a single electrolyzer cell as a function of CO mol per cent (mol%) in the CO2/CO co-feed, measured for various applied current densities in Cu-based cell-2. Production rates are shown forahydrogen,bethylene,cethanol anddn-propanol. Electrolysis was conducted in single-cell experiments deploying only the Cu-based electrolyzer denoted as cell-2. The total volumetric flow of co-feed mixtures was kept constant at 50 mL min−1throughout all experiments, while the CO concentration was gradually increased. Displayed values represent the average and error bars the standard deviation of at least 2 independent measurements. Figure 2 displays the production rates of the four most prominent reaction products, i.e., hydrogen, ethylene, ethanol, and n-propanol as a function of CO mol% in the CO 2 /CO co-feed and of applied current density. While the absolute volumetric flow of the gas feed was kept constant at 50 mL min -1 , we have varied its composition by adjusting the individual flow rates of CO 2 and CO that were mixed prior to entering cell-2. Figure 2a shows a profound effect of CO in the co-feed on the production of hydrogen. For CO-lean feeds, an increase in CO raised H 2 production, as well, before H 2 production rates dropped for CO-rich co-feeds. The molar CO concentration associated with the maximum H 2 production depended on the applied current density. While for low current densities such as 100 or 200 mA cm -2 the turning point was at 66 mol% CO , larger current densities showed the transition at 50 mol% CO (300 and 400 mA cm -2 ), or even at 34 mol% CO (500 to 700 mA cm -2 ). The single-maximum pattern of hydrogen production appears surprising, as the total carbon content in the electrolyte monotonically drops with more CO due to the vastly lower solubility of CO versus CO 2 . So, CO x surface coverages should monotonically decline, as well. For the production rate of ethylene, shown in Fig. 2b, a distinctly different trend was apparent. Here, increasing CO mol% improved the ethylene production rate. Note that this improvement was most significant up to a co-feed composition of 50 mol% CO , beyond which it plateaued. The production rates of ethanol and n-propanol, Fig. 2c, d , showed unusually sharp enhancements with rising molar CO mol% in the co-feed. In contrast to the trends observed for ethylene, the beneficial effect on production rate was most pronounced past 50 mol% CO approaching pure CO gas feed. Production rates of other compounds such as formate, acetate and ally alcohol can be found in Supplementary Fig. 3 . The trend for allyl alcohol generally agrees with the behavior observed for other alcohols, whereas formate production was suppressed by raising CO content in line with expectations. Fig. 2: Influence of CO 2 /CO co-feed composition on production rates observed for electrolysis in single-cell experiments of cell-2. Production rates of key products using a single electrolyzer cell as a function of CO mol per cent (mol%) in the CO 2 /CO co-feed, measured for various applied current densities in Cu-based cell-2. Production rates are shown for a hydrogen, b ethylene, c ethanol and d n-propanol. Electrolysis was conducted in single-cell experiments deploying only the Cu-based electrolyzer denoted as cell-2. The total volumetric flow of co-feed mixtures was kept constant at 50 mL min −1 throughout all experiments, while the CO concentration was gradually increased. Displayed values represent the average and error bars the standard deviation of at least 2 independent measurements. Full size image To better appreciate the effect of CO in the feed, let us consider the kinetic enhancements of individual C 2+ production rates on a relative scale to pure CO 2 feeds: CO in the feed has the most significant effect on PrOH production, showing a 4x increase in rate, followed by a 2-3x increase of EtOH production and finally 2x increase in C 2 H 4 production. This sharp enhancement of C 2+ oxygenate production under CO-rich feed conditions is also reflected by the dramatically larger FE values obtained for pure CO feed (CORR) compared to pure CO 2 feed (CO 2 RR), Supplementary Fig. 4 . These enhancements can be explained mechanistically by enhanced cross-coupling CO dimerization rates on the surface of the Cu catalyst [20] . The combined presence of CO 2 and CO gas in the feed offers new C-C coupling pathways between two adsorbed CO surface species derived from both CO 2 and CO on two distinct, non-scrambling Cu surface sites, in line with the multi-site hypothesis on Cu catalysts [20] , [42] . Kinetic analysis of CO 2 RR and CORR of CO 2 /CO feeds To gain a better understanding of the origin of the CO dependence of the production rates, we tracked the applied cathode potentials as well as the CO consumption during co-feed experiments. 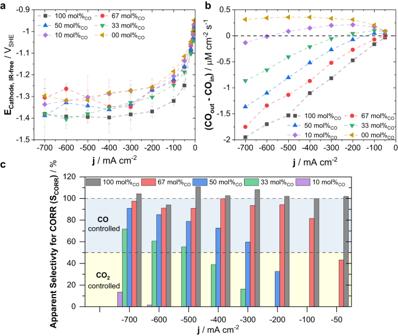Fig. 3: Electrode potential and CO conversion under CO2/CO co-feed conditions in single-cell experiments of cell-2. aIR-corrected cathode polarization curves as a function of applied current density for various investigated co-feed compositions.bThe net CO flux, COnet flux, defined as the difference in the molar CO influx, COin, and molar CO outflux, COout, plotted versus the applied current density and co-feed composition.cApparent selectivity for CORR, denoted SCORR, as a function of applied current density and co-feed composition. SCORRwas defined as the ratio between the electrocatalytic CO consumption rate (COconsumption= –COnet flux) and the theoretically required molar CO consumption rate to produce all C2+species by CORR. Colored areas indicate regions controlled by the respective primary reactant used in the production of C2+species, either CO or CO2, dependent on the absolute value of SCORR. Electrolysis was conducted in single-cell experiments deploying only the Cu-based electrolyzer denoted as cell-2. The total volumetric flow of co-feed mixtures was kept constant at 50 mL min−1throughout all experiments, while the CO concentration was gradually increased. Displayed values represent the average and error bars the standard deviation of at least 2 independent measurements. Figure 3a shows IR-free cathode polarization curves obtained for experiments at varying CO feed concentrations. Evidently, cathode overpotentials (E cathode, IR free ) during electrolysis in pure CO 2 and in small molar CO co-feeds of 10 mol% remained near −1.3 V SHE at a current density approaching 700 mA cm –2 . In contrast, the required cathode potentials shifted to –1.4 V SHE for the case of a pure CO feed, possibly pointing to concentration overpotentials due to lower CO solubility. Fig. 3: Electrode potential and CO conversion under CO 2 /CO co-feed conditions in single-cell experiments of cell-2. a IR-corrected cathode polarization curves as a function of applied current density for various investigated co-feed compositions. b The net CO flux, CO net flux , defined as the difference in the molar CO influx, CO in , and molar CO outflux, CO out , plotted versus the applied current density and co-feed composition. c Apparent selectivity for CORR, denoted S CORR , as a function of applied current density and co-feed composition. S CORR was defined as the ratio between the electrocatalytic CO consumption rate (CO consumption = –CO net flux ) and the theoretically required molar CO consumption rate to produce all C 2+ species by CORR. Colored areas indicate regions controlled by the respective primary reactant used in the production of C 2+ species, either CO or CO 2 , dependent on the absolute value of S CORR . Electrolysis was conducted in single-cell experiments deploying only the Cu-based electrolyzer denoted as cell-2. The total volumetric flow of co-feed mixtures was kept constant at 50 mL min −1 throughout all experiments, while the CO concentration was gradually increased. Displayed values represent the average and error bars the standard deviation of at least 2 independent measurements. Full size image As our co-feeding experiments introduced two distinct reactants, i.e., CO 2 and CO, we set out to quantify whether and how the shift in C 2+ production rates with CO mol% correlated with a shift from predominantly CO 2 -controlled electroreduction to a predominantly CO-controlled one. For that purpose, we measured the CO outflux (area-normalized molar outflow rates) out of the electrolyzer at various co-feed compositions, Supplementary Fig. 5 . Considering the large stoichiometric excess of reactants in the input feed, CO conversion was incomplete for all investigated co-feeds. Higher CO mol% in the feed led to higher molar CO outflux, CO out , from the electrolyzer. However, the decrease in CO out with larger current density was significantly more pronounced for CO-rich co-feeds, suggesting a larger relative consumption thereof. Taking the difference between the molar CO influx, CO in , and the molar CO outflux during electrolysis, we derived the net CO flux , defined as CO net flux = (CO out - CO in ), as function of applied current and co-feed composition, Fig. 3b . In this plot, positive and negative values of CO net flux denote a catalytic net production and net consumption of CO, respectively. Generally, both higher CO mol% in the feed and larger current density led to increasing CO consumption, i.e., more negative values of CO net flux . For CO mol% <= 50 in the feed, there appeared a critical current density, beyond which net CO production turned into net CO consumption (10, 33 and 50 mol% CO at 500, 200 and 100 mA cm -2 , respectively). For CO mol% > 50, only net CO consumption was apparent over the entire range of current density. This data allowed us to estimate what fraction of the produced C 2+ species can be accounted for by an exclusive CORR pathway. To do that, we considered the apparent CO reduction reaction selectivity , S CORR , defined as the ratio of the experimental CO consumption rate, CO consumption = –CO net flux and the theoretical CO demand that is required for the combined experimental C 2+ production rate, according to: 
    S_CORR=CO_consumption/∑_i(ṅ_i ν_i) · 100%
 (1) where \({\nu }_{i}\) and \({\dot{n}}_{i}\) denote the number of carbon atoms in species i and its molar production rate, respectively. Figure 3c plots S CORR versus the co-feed compositions and the applied current density. Both CO mol% in the feed and applied current density control S CORR , with S CORR approaching 100% with larger applied current density or with rising CO mol%. As expected, a pure CO feed showed a S CORR of 100% at all currents, agreeing with the conditions of CO being the only reactant. Importantly, sustained S CORR values near 100% were evident for 67 mol% CO feed and currents as low as 200 mA cm −2 . This observation suggests that under conditions of 67 mol% CO and 200 mA cm -2 essentially all C 2+ product formation can be accounted for by the reduction and dimerization of CO gas (prevalent CORR). This kinetic effect arises because the catalytically effective gas composition at the catalyst-electrolyte-interface differs from the bulk gas feed composition. It is a consequence of the preferential acid-base reaction of CO 2 in CO 2 /CO co-feeds with catalytically generated OH − [18] , [19] . This acid-base reaction increases the effective CO concentration for a given CO 2 /CO co-feed, and this will become more severe at a larger current. Using S CORR , we split the catalytic co-feed reduction kinetics into a CO-controlled regime (S CORR > 50%) and a CO 2 -controlled one (S CORR < 50%), see colored regions in Fig. 3c , which deconvolutes the overall reduction reactivity. Carbon Selectivity of C 2+ production under CO 2 /CO co-feeds Rising CO concentration in CO 2 /CO co-feeds sharply enhances the total production rates of C 2+ species (Fig. 2 ). In part, this influence could be explained by the reduced number of electrons required to produce C 2+ species from the CORR pathway, see Supplemental Discussion 1 . However, charge stoichiometry falls short of the 2 to 4-fold experimental increase shown in Fig. 2 . This is manifested in the single feed experiments CO 2 RR and CORR in Supplementary Fig. 4 that showed drastically larger FE values for C 2+ species in CORR experiments: In particular, the FE values of alcoholic oxygenates showed sharp increase under CORR compared to CO 2 RR [14] , [16] . We hypothesize that the sharp rise in the C 2+ production must originate from a change in surface catalytic selectivity associated with an enrichment of CO gas in the feed inside the electrolyzer, and associated with a changed surface coverage of CO at the Cu catalyst. Accurate calculation of faradaic product selectivity requires knowledge of the electron transfer numbers, which, however, are not known for co-feeding. This is why, for the purpose of a mechanistic discussion, we calculated a carbon selectivity of species i, CS i , (see Supplementary Fig. 6 ) defined as the ratio between the carbon atom flux into an individual C 2+ species i and the total carbon atom flux into all C 2+ products. CS_i=ṅ_iν_i/∑_i(ṅ_i ν_i)· 100%
 (2) Here, \({\dot{n}}_{i}\) and \({\nu }_{i}\) denote the molar production rate of species i and the number of carbon atoms in species i, respectively. CS i reveals changes in mechanistic reaction pathways for different co-feeds and currents and can be compared to kinetic modeling results. More detailed information on CS i is given in the Supplemental Discussion 1 . In Supplementary Fig. 6 , CS ethylene showed a maximum at 33 CO mol% and decreased at higher CO mol% in the feed. Above 10 mol% CO , CS EtOH rose gradually by ca. 10 percentage points, and so did CS PrOH . Evidently, higher CO mol% favor formation of oxygenates. While the applied current density showed a minor effect on CS Ethylene , the production of either alcohol was profoundly affected: Higher currents favor the production of EtOH over PrOH. Mechanistically, this can be rationalized by a lower surface coverage of CO that makes formation of C 3 products less likely, as concluded in prior experiments of pure CO feeds at varying partial pressures [12] , [13] , [44] , [45] , [46] . A more detailed mechanistic discussion of the observed trends in CS i values under CO 2 /CO co-feeds is provided in the Supplemental Discussion 2 . Operation of a two-cell, tandem system for enhanced production rates and energy efficiency of C 2+ compounds After we had deconvoluted and rationalized the increase in overall C 2+ production rates under controlled CO 2 /CO co-feed electrolysis, we moved to assemble, operate, and analyze the first complete low-temperature, coupled CO 2 tandem electrolyzer cell system excluding intermediate processing steps. Unlike tandem catalyst designs [20] , tandem cell designs allow for individually optimized active sites and electrolysis conditions for each step. We generated CO-rich co-feeds in “Cell-1” using a neutral-pH, zero-gap electrolyzer with a Ni-N-C catalyst-based Gas Diffusion Electrode (GDE) [43] . The use of the CO 2 -to-CO electrolyzer as cell-1 allowed precise control over the resulting mixed CO 2 /CO exit gas composition (equivalent down-stream to the CO 2 /CO co-feed into cell−2) via two control parameters, that is the applied current density and the CO 2 feed rate. As operating conditions of cell-1, we selected 200 mA cm −2 and near-100% FE CO including only minute amounts of H 2 to achieve a controlled mixed of predominantly CO 2 /CO exit steam out of cell-1. Supplementary Fig. 7 shows how the FE CO affects the absolute CO production rate as a function of the applied current density of cell-1. At the chosen operating point, cell-1 generates about 7.6 ml CO min -1 . To ensure stable performance of cell-1, we monitored the experimental FE CO and cell potential over the electrolysis time of 12 hours at 200 mA cm −2 , shown in Supplementary Fig. 8 . We thereby convinced ourselves that the FE CO value remained at near-unity without changes in the cell potential. Since the CO 2 flow rate into cell-1 controls the molar CO 2 /CO ratio of the exit steam, we have also investigated the effect of CO 2 flow rate. We chose (i) a flow rate of 50 ml min −1 corresponding to the total flow rate of the co-feed tests above, and (ii) a reduced CO 2 flow rate of 30 ml min −1 to enrich the exit flow in CO further. In cell-1 the CO 2 flow of 50 mL min −1 was converted to a gas mixture (co-feed) of CO 2 and CO with 18 mol% of CO and a total volumetric flow rate of 42 mL min −1 , whereas a CO 2 input of 30 mL min −1 resulted in an exit flow of 22 mL min −1 with 35 mol% of CO. 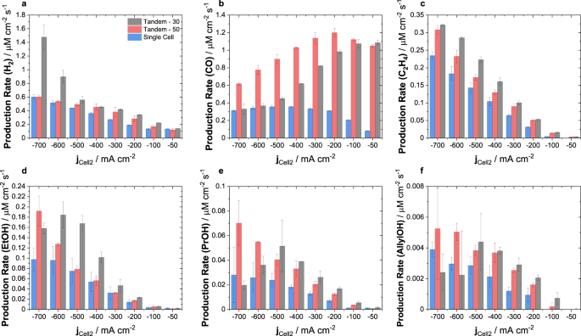Fig. 4: Product production rate comparison of tandem electrolyzer cell cascade (cell-1 and cell-2) versus a single electrolyzer cell. Production rate ofahydrogen,bcarbon monoxide,cethylene,dethanol,en-propanol, andfallyl alcohol as a function of current density applied to cell-2. Values given in the legend correspond to the volumetric flow of CO2introduced to the tandem system. In the tandem configuration, cell-1 has been continually operated at a current density of 200 mA cm−2while the current density applied to cell-2 has been varied. For both cells the active geometric surface area is 5 cm2. The single-cell refers to CO2RR experiments using only cell-2 of the reaction cascade at a CO2volume flow of 50 mL min−1. Displayed values represent the average and error bars the standard deviation of at least 2 independent measurements. Figure 4 compares the catalytic production rates of the tandem system versus the reference single-cell CO 2 RR (using cell-2) as a function of the applied current density of cell-2. The investigated CO 2 flow rates of 50 mL min −1 and 30 mL min −1 are denoted as Tandem-50 and Tandem-30 , respectively, the reference is denoted as Single Cell . In good agreement with our previous experiments, hydrogen production slightly increased with more CO in the co-feed between cell-1 and cell-2, Fig. 4a . Tandem-30 showed a larger H 2 production rate than Tandem-50, consistent with its larger CO mol% in the exit of cell-1. While Tandem-50 matched the H 2 production rate of the single-cell experiment at 700 mA cm −2 , H 2 rate of Tandem-30 increased rapidly at larger current densities, most likely due to reactant transport limitation. CO production rates of Tandem-50/30 at 50 mA cm −2 , Fig. 4b , are controlled by CO production of cell-1. CO rates of Tandem-30 declined steadily approaching the Single Cell, while CO rates of Tandem-50 showed a maximum at 200 mA cm −2 before declining. Ethylene rates , Fig. 4c , were significantly enhanced (up to 50% at 500 mA cm −2 ) for the Tandem case over the entire current density range. A similar behavior was seen in the EtOH production rates , Fig. 4d , with space-time yield enhancements of up to 100% at 700 mA cm −2 . Likewise, production rates of C 3 compounds , i.e., PrOH and AllylOH, Fig. 4e, f , showed more than 100% enhanced production rates at 700 mA cm −2 in tandem configuration, with Tandem-30 suffering from mass transport limitations. Fig. 4: Product production rate comparison of tandem electrolyzer cell cascade (cell-1 and cell-2) versus a single electrolyzer cell. Production rate of a hydrogen, b carbon monoxide, c ethylene, d ethanol, e n-propanol, and f allyl alcohol as a function of current density applied to cell-2. Values given in the legend correspond to the volumetric flow of CO 2 introduced to the tandem system. In the tandem configuration, cell-1 has been continually operated at a current density of 200 mA cm −2 while the current density applied to cell-2 has been varied. For both cells the active geometric surface area is 5 cm 2 . The single-cell refers to CO 2 RR experiments using only cell-2 of the reaction cascade at a CO 2 volume flow of 50 mL min −1 . Displayed values represent the average and error bars the standard deviation of at least 2 independent measurements. Full size image The experimental performance of the tandem systems are in good agreement with our CO 2 /CO co-feeds results. Tandems showed a sharp increase in C 2+ production rates over the single-cell CO 2 RR experiments. While C 2+ production rates of Tandem-30 were superior to Tandem-50, consistent with the larger CO concentration in the co-feed to cell-2, clear signs of mass transport limitation were apparent when exceeding a current density of 500 mA cm −2 , reflected in a rising H 2 rate and a declining C 2+ rate. Note that the extent of the decrease in C 2+ rates at large current density followed the order of PrOH/AllylOH>EtOH>C 2 H 4 suggesting that C 3 compounds are more susceptible to the insufficient reactant transport. This behavior fits well with our previous observation in single-cell experiments that showed that C 3 production rates were particularly sensitive to CO depletion in the gas feed. In order to provide a direct comparison of product productions in the tandem experiments (18 mol% CO for Tandem-50, and 35 mol% CO for Tandem-30) and the CO 2 /CO co-feed experiments, we overlaid their production rates in Supplementary Fig. 9 . This revealed some unexpected, yet important kinetic discrepancies: In either tandem experiment, the observed production rates suggested a higher CO mol% in the co-feed to cell-2 than inferred from the overlaid co-feed single-cell experiments. This trend is also reflected in the C 2+ product carbon selectivity comparisons in Supplementary Fig. 10 . With larger current densities, this seeming CO-enrichment becomes progressively more pronounced. To explain this observation, we recall the lower actual tandem feed rates of 42 mL min −1 and 22 mL min −1 for Tandem-50 and Tandem-30, respectively, compared to 50 mL min −1 for the single cell case. This difference in available CO 2 becomes clearer in a direct comparison of the molar reactant flow to cell-2 under the various conditions, see Supplementary Fig. 11 . As a result of this, at a given OH - generation (given current density), the lower molar CO 2 flow into cell-2 results in a larger share of CO 2 being depleted. This enhances the effective CO concentration near the electrode, and results in a product pattern resembling a higher bulk mol% CO . The technological application of the tandem concept ultimately requires an acceptable overall energy efficiency , henceforth denoted EE . Estimation of EE values in a tandem system requires power-in /power out consideration of both cells of the reaction cascade. Equation ( 3 ) defines the EE as the ratio between the rate of chemical energy stored in products based on their higher heating values (HHV) and the total electrical input power introduced to the electrolyzer system. EE_i(HHV)=ṅ_i HHV_i/I_Cell1*E_Cell1+I_Cell2*E_Cell2*100%
 (3) In Fig. 5 , we compare the performance of the single-cell and tandem system experiments with particular focus on the electrical power consumption, energy efficiency, and system characteristics. 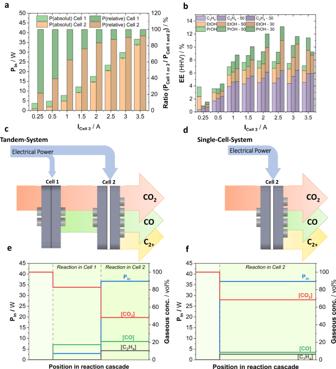Fig. 5: Efficiency and system characteristics comparison between single-cell and tandem experiments. aTotal input Power, Pin, as function of applied current to cell-2 deconvoluted in absolute and relative terms into the individual contributions of cell-1 and cell−2 during tandem experiments with CO2input flow of 50 mL min−1.bEnergy efficiency for C2H4, EtOH and n-PrOH based on their higher heating value (HHV) as a function of applied current for single-cell and tandem experiments. Tandem experiments are labeled in the legend with the respective input flow of CO2(30 or 50 mL min−1).c,dSchematic illustrations of c the tandem electrolyzer cell system and d single-cell system with arrows indicating the flow of products and reactants, CO2, CO and C2+, as well as the distribution of electrical power across the coupled electrochemical cells.e,fDistribution profiles of total power input and concentrations of CO2, CO and C2H4within the reaction cascade for e tandem experiments with 50 mL min−1CO2feed and f single-cell experiments. In the tandem configuration, cell-1 has been continually operated at a current density of 200 mA cm−2while the current density applied to cell-2 has been varied. For both cells the active geometric surface area is 5 cm2. Displayed error bars represent the standard deviation of at least 2 independent measurements. Figure 5a deconvolutes the electrical input power, P in , of the Tandem-50 system in terms of cell-1 and cell−2 in absolute and relative terms. As cell-1 was operated at constant current and cell voltage, absolute P in of cell-1 remained constant, while P in of cell-2 strongly increased. This has important implications for the relative P in balance between the two cells: At low currents applied to cell-2, total P in is clearly dominated by cell-1, later by cell−2 increasing to over 90% at 3.5 A. This is because of the higher applied currents and cell resistances of the 1-gap design of cell−2 compared to the zero-gap design of cell-1. Fig. 5: Efficiency and system characteristics comparison between single-cell and tandem experiments. a Total input Power, P in , as function of applied current to cell-2 deconvoluted in absolute and relative terms into the individual contributions of cell-1 and cell−2 during tandem experiments with CO 2 input flow of 50 mL min −1 . b Energy efficiency for C 2 H 4 , EtOH and n-PrOH based on their higher heating value (HHV) as a function of applied current for single-cell and tandem experiments. Tandem experiments are labeled in the legend with the respective input flow of CO 2 (30 or 50 mL min −1 ). c , d Schematic illustrations of c the tandem electrolyzer cell system and d single-cell system with arrows indicating the flow of products and reactants, CO 2 , CO and C 2+ , as well as the distribution of electrical power across the coupled electrochemical cells. e , f Distribution profiles of total power input and concentrations of CO 2 , CO and C 2 H 4 within the reaction cascade for e tandem experiments with 50 mL min −1 CO 2 feed and f single-cell experiments. In the tandem configuration, cell-1 has been continually operated at a current density of 200 mA cm −2 while the current density applied to cell-2 has been varied. For both cells the active geometric surface area is 5 cm 2 . Displayed error bars represent the standard deviation of at least 2 independent measurements. Full size image Figure 5b plots the EE of C 2 H 4 , EtOH and PrOH in Tandem-50 and Tandem-30 versus the single-cell design. While at low currents the single-cell system shows competitive C 2+ EE values, at larger currents > 1 A tandem designs sharply outperform the single-cell system. In particular, the Tandem-30 experiments shows a strongly enhanced total absolute C 2+ EE of up to 13%. We then analyzed the individual EE of C 2 H 4 , EtOH and PrOH as a function of total P in for each electrolyzer design in Supplementary Fig. 12 . The tandem systems showed relative enhancements in C 2+ EE values of up to 100% over a broad operation range, in particular Tandem-50 at high C 2+ productivities and large power inputs. At low power input, the productivity of the tandem system was dominated by cell-1 reflected in the high EE for CO and low EE for H 2 in comparison to the single-cell system shown in Supplementary Fig. 13 . In addition to the advantages for EE, we also observed a more efficient reactant utilization described by the single pass carbon efficiency, SPCE. When directly comparing the single-cell system to the tandem-system, the SPCE nearly doubled from 17% to 30–35% depending on the applied current, see Supplementary Fig. 14 . The increase in SPCE was larger than can be expected by a simple consideration of the additional operation of cell-1 suggesting the inherent benefit of tandem operation. A more detailed discussion can be found in the Supplementary Information of this work. Apart from the electrochemical performance differences, tandem electrolyzer systems also differ from a single-cell system in terms of some of their process characteristics. As the single-cell system deploys only one single reactor, the total input power, the CO 2 consumption, and product generation occur at the same physical location, schematically depicted in Fig. 5d . This results in a single-stepped experimental concentration and power profile, as given for 700 mA cm −2 in Fig. 5f . By contrast, in the tandem system the total input power splits into two reactors and the conversion of CO 2 occurs along a reaction cascade, schematically depicted in Fig. 5c . Consequentially, the experimental concentration and power profile at 700 mA cm −2 (cell-2), given in Fig. 5e , reveals two distinct steps. In summary, we have designed, assembled, and analyzed the first full low-temperature tandem electrolyzer cell system designed for an efficient electrochemical CO 2 reduction to C 2+ products, such as Ethylene, EtOH, and PrOH. The tandem design consisted of two low-temperature electrolyzer cells in series, which enabled a catalytic reaction cascade of the reaction of CO 2 to mixed CO 2 /CO streams in cell-1, coupled to the reaction of mixed CO 2 /CO feeds to C 2+ products in cell-2. We demonstrated that the tandem system strongly enhanced production rates of C 2+ compounds compared to the use of a conventional singe-cell system. We also provided evidence that the additional power input required to operate the tandem system was comperatively minor thanks to the drastically lower energetic demand of the CO 2 -to-CO electrolyzer cell-1. Consequentially, the proposed tandem system allowed for an increase in individual EE of C 2+ species compared to the conventional single-cell system. Electrochemical cell and electrode preparation Depending on the target product of electrolysis, electrochemical tests were performed using two different cell geometries. In the case of CO 2 -to-CO reduction, a “zero-gap” cell was used shown in Supplementary Fig. 2a , referred to as cell-1. For the reduction of either CO 2 or CO, or co-feed mixtures of the two to produce C 2+ species a “one-gap” cell was used, shown in Supplementary Fig. 2b , referred to as cell-2. Details on cell-1 The Ni-N-C catalyst used in this work was synthesized through thermal carbonization of a Ni-imidazolate according to a previously established procedure. In short, to an aqueous solution of Ni(NO 3 ) 2 and imidazole, a NaOH solution was added dropwise. After overnight stirring, the precipitate was filtered, washed, and freeze-dried. This catalyst precursor material was then carbonized by thermal treatment in N 2 atmosphere at 800 °C. The crude product was acid-washed at 80 °C in H 2 SO 4 , followed by rinsing with water to pH-neutral and freeze-drying to obtain the final catalyst powder [43] . For the preparation of the cathode GDE, 55 mg as-prepared Ni-N-C catalyst, 195 mg Sustainion solution (Dioxide Materials, 5 wt% Sustainion in ethanol solution), 100 μL DI-water and 2900 μL isopropanol were mixed and sonificated using a sonifer horn for 15 mins. Afterwards, the prepared ink was sprayed coated at 60 °C onto 5 cm 2 of the micro porous side of a commercial gas diffusion layer provided by DeNora (GDL2). As electrochemical cell, a membrane electrode assembly type electrolyzer setup was deployed for the CO 2 to CO conversion. An exploded-view of the electrolyzer system is given in Supplementary Fig. 2a . The catalyst-coated cathode GDL, membrane (Sustainion membrane X37-50 RT, Dioxide material), and the anode (5 cm 2 , commercial IrO 2 -GDE supplied from Dioxide Materials) were assembled layer by layer including PTFE gaskets (thickness: 200 microns; window size: 5c m 2 ) to guarantee for leak-tightness. Finally, all layers were compressed between the electrolyzer endplates, which served as flow fields and current collectors. For catalytic tests involving cell-1, an aqueous solution of 0.1 M KHCO 3 electrolyte was used on the anode side only and constantly recycled at a volumetric flow rate of 20 mL min −1 . On the cathode, a humidified stream of CO 2 was introduced by a mass flow controller at a rate of 25 mL min −1 . After the reaction in cell-1, the product stream, composed mainly of CO and unreacted CO 2 , was introduced as reactant gas feed to the cathode GDE of cell-2. Details on cell-2 As anode material Ni foam (Fraunhofer IFAM, thickness of 0.45 mm) was placed inside the flow field of the anode Titanium endplate (Dioxide materials). For the preparation of the cathode GDE a sintered PTFE membrane (Elringklinger, thickness of 0.5 mm) was used as substrate and coated by spray-painting with a dispersion of commercial spherical Cu particles (Sigma-Aldrich, 40–60 nm) and PTFE particles (Sigma-Aldrich, 1 μm) in ethanol. The relative content of PTFE particles was adjusted to achieve a final loading of 20 wt.% in relation to the combined loading of Cu and PTFE particles on the substrate. The absolute loading of Cu particles on the PTFE substrate was controlled by the volume of the catalyst dispersion used during the spray-painting process and fixed at 3.0 mg cm −2 throughout the whole study. When assembling the electrolysis cell, the Cu-PTFE GDE is fixed to the cathode Titanium endplate with a conductive Cu tape to enable electronic contacting of the catalyst layer. Silicon gaskets of 0.5 mm in thickness and a cut-out window of 5 cm 2 were used to expose 5 cm 2 of the electrode as geometric active area and guarantee a leak-free operation during catalytic testing. An aqueous solution of 1.0 M KHCO 3 with a volume of 500 mL each was deployed as anolyte and catholyte solution. In the cathode compartment, a custom-designed flow field composed of PEEK and a thickness of 1.0 mm was deployed. The anode and cathode compartments of the electrochemical cell were separated by an anion exchange membrane (Selemion, AMV). Electrochemical setup For electrochemical testing the electrolysis cell was embedded in the teststand depicted in Supplementary Fig. 2c that allowed careful control over pressure levels, as well as gas and electrolyte flow rates. Mass flow controllers (Bronkhorst) were used to accurately adjust the flow of all gases (N 2 , CO, CO 2 ). The reactant gas feeds, CO 2 and CO pure feeds or gas mixtures of the two, were introduced at a total constant rate of flow of 50 mL min −1 . The anolyte and catholyte were constantly recirculated through the respective compartments of the cell by membrane pumps (KNF, SIMDOS 10) at a constant flow of 50 mL min −1 . Additionally, a dead volume filled with gas is induced on the inlets and outlets of the membrane pumps to mitigate their inherent pulsation during operation. The cell was operated with an overpressure on the liquid side of the cathode GDE. Here, the differential pressure across the cathode was set to 100 mbar by adjusting the absolute pressure of the cathode gas side to 1.300 bar and the absolute pressure of the catholyte reservoir headspace to 1.400 bar by use of back pressure regulators (Bronkhorst). Electrochemical measurement protocol Electrochemical characterization for cell-2 was carried out according to a preset measurement protocol comprising three successive measurement techniques: Firstly, galvanostatic steps in current density, secondly cyclovoltammetry (CV) and finally galvanostatic electrochemical impedance spectroscopy (GEIS). All electrochemical data that show error bars represent the mean values and standard deviation obtained from at least two independent samples. Galvanostatic current density steps Here, after an initial equilibration time of 20 min at open circuit potential (OCP), the cathodic current density was increased stepwise as follows: 50, 100, 200, 300, 400, 500, 600 and finally 700 mA cm −2 . After the 700 mA cm −2 current density step, the current was decreased again, retracing the previous steps in the opposite direction towards a final current density of 50 mA cm −2 . During the whole procedure, each of the set current density steps was kept constant for a period of 20 min before moving towards the next value. Cyclovoltammetry (CV) After completion of the galvanostatic current density steps, CVs were conducted in a potential window of 100 mV (−0.600 to −0.700 V Ag/AgCl ). Within this potential window 5 CVs were conducted at a constant scan rate before increasing the scan rate and performing 5 CVs again. This procedure was performed sequentially for scan rates of 1, 2, 5, 10, 20, 50, 100, 200, 500, 700, 1000, 1500 and 2000 mV s −1 . Galvanostatic electrochemical impedance spectroscopy (GEIS) In the final step, GEIS measurements were conducted at 1, 10, 20, 50, 100, 200, 300, 400, 500, 600, and 700 mA cm −2 of absolute cathodic current. The frequency was varied between 500 kHz and 100 mHz and the amplitude of the interference signal was set to 10% of the respective current density value at which the GEIS measurement was carried out. Quantification of products All data that show error bars represent the mean values and standard deviation obtained from at least two independent samples. Gaseous products After electrochemical reaction in the electrolyzer the outgoing gas stream was mixed with a constant flow of N 2 as an internal standard (16 mL min −1 ) and CO 2 (150 mL min −1 ) that has been purged through the headspace of the catholyte compartment in order to collect gaseous products that were released at the catholyte side during operation. This mixture of gases was introduced into a gas chromatograph (Shimadzu, GC 2014 series) in the following denoted as GC. The GC was equipped with a thermal conductivity detector (TCD) used in the quantification of H 2 and N 2 concentrations, as well as a flame ionization detector (FID) that was used for quantification of methane, ethylene and CO. For the detection of CO by the FID a methanizer has been used for the thermal reduction of CO to CH 4 prior to its detection. Determination of the absolute volumetric flow after electrolysis has been conducted based on changes in the concentration of N 2 standard as detected by the TCD. Liquid products During electrolysis, aliquots of the catholyte have been collected after 20 min of reaction time at constant current. These aliquots were analyzed for their content of alcohols by liquid injection gas chromatography (Shimadzu, GC 2010 series) equipped with an FID. Furthermore, a high-performance liquid chromatograph (Agilent, 1200 series) equipped with a refractive index detector has been deployed for quantification of carbonic acids and their respective salts.